De novo TBR1mutations in sporadic autism disrupt protein functions Next-generation sequencing recently revealed that recurrent disruptive mutations in a few genes may account for 1% of sporadic autism cases. Coupling these novel genetic data to empirical assays of protein function can illuminate crucial molecular networks. Here we demonstrate the power of the approach, performing the first functional analyses of TBR1 variants identified in sporadic autism. De novo truncating and missense mutations disrupt multiple aspects of TBR1 function, including subcellular localization, interactions with co-regulators and transcriptional repression. Missense mutations inherited from unaffected parents did not disturb function in our assays. We show that TBR1 homodimerizes, that it interacts with FOXP2, a transcription factor implicated in speech/language disorders, and that this interaction is disrupted by pathogenic mutations affecting either protein. These findings support the hypothesis that de novo mutations in sporadic autism have severe functional consequences. Moreover, they uncover neurogenetic mechanisms that bridge different neurodevelopmental disorders involving language deficits. Autism spectrum disorders (ASD) are estimated to affect 1 in 88 individuals and are characterized by a classic triad of symptoms, which include impairments in social interactions, deficits in communication and a tendency for repetitive stereotyped behaviours (CDC 2012). Inherited genetic variants may account for 40% of the risk for developing ASD [1] , but as is typical for complex traits, the effect of individual common variants is small [2] . In recent years, next-generation sequencing in ASD probands and their families has revealed that rare and private genetic variants play a major role in the aetiology of the disorder. These studies suggest that loss-of-function mutations within any of a large number of different genes may be sufficient to cause ASD. For some genes, such as AMT , PEX7 and SYNE1 , the pathogenic mechanism involves complete gene knockout through rare inherited mutations, in a homozygous or compound heterozygous state. For other genes, it is proposed that de novo loss-of-function mutations disturbing one gene copy are responsible for sporadic severe cases of ASD [3] , [4] , [5] , [6] , [7] , [8] . Six genes— CHD8 , DYRK1A , GRIN2B , PTEN , TBR1 and TBL1XR1 —have been observed to harbour de novo mutations in multiple unrelated probands, strongly suggesting that heterozygous disruption of any one of these genes is sufficient to cause ASD. It is estimated that mutations at these loci may account for 1% of sporadic cases [8] . TBR1 is of particular interest, because it encodes a neuron-specific transcription factor of the T-box family. T-box proteins have diverse biological roles [9] and haploinsufficiency of this class of regulatory protein has already been established as a cause of human disease [10] —for instance, ulnar-mammary syndrome and Holt–Oram syndrome are caused by haploinsufficiency of TBX3 and TBX5 , respectively [11] , [12] , [13] . TBR1 has established roles in patterning of the central nervous system, including regulation of neuronal identities during cortical development [14] . It is striking that among the small number of known TBR1 targets, three— RELN , GRIN2B and AUTS2 —have been implicated in ASD [3] , [7] , [8] , [15] , [16] , [17] , [18] . Of particular interest, GRIN2B is one of the six genes mutated recurrently in ASD. TBR1 , RELN , GRIN2B and AUTS2 may therefore form part of a molecular network important for cortical development that is recurrently mutated in ASD. Moreover, there are data to suggest that the TBR1 protein may be a potential interaction partner of the forkhead transcription factor FOXP2 (ref. 19 ), another key regulator of central nervous system development and function [20] . In the mammalian cortex, TBR1 and FOXP2 show striking similarities in expression pattern [21] , [22] , [23] , [24] , raising the possibility that they cooperate to regulate gene networks in deep layer cortical neurons, and other neural sites of co-expression. Mutations in FOXP2 cause a rare disorder characterized by problems with sequencing speech, and impairments in expressive and receptive language affecting spoken and written domains [20] . Given that communication deficits are a core feature of ASD, it is plausible that TBR1 and FOXP2 belong to a shared molecular network, which goes awry in different neurodevelopmental disorders involving impaired speech and/or language skills. The recurrence of de novo TBR1 mutations in sporadic ASD suggests that the identified mutations are likely to be pathogenic. Nonetheless, functional experiments in model systems are essential to determine the precise effect of mutations on protein function and provide insight into the molecular mechanisms of the disorder [25] . Follow-up of findings from genetic studies of ASD is beginning to uncover the relevant gene networks and biological pathways [8] , [23] , [26] , [27] , [28] . For example, two recent independent reports highlight network clusters of ASD risk genes that are important in mid-fetal brain development and glutamatergic neuronal function [23] , [28] . In the present study, we perform the first functional characterization of de novo TBR1 mutations identified in sporadic cases of ASD, assessing their impact on multiple aspects of protein function including protein expression, subcellular localization, transcriptional repression and protein–protein interactions. We compare the functional consequences of these de novo mutations with rare inherited TBR1 mutations of uncertain clinical significance, also found in probands with sporadic ASD. Moreover, we define functional interactions between TBR1 and FOXP2 proteins, assessing the impact of aetiological mutations in each protein on these interactions. This work demonstrates how functional analyses of de novo mutations from next-generation sequencing can be used to define and expand a key molecular network involved in neurodevelopmental disorders. TBR1 mutations in sporadic ASD Four de novo TBR1 coding mutations have been reported in sporadic ASD cases ( Fig. 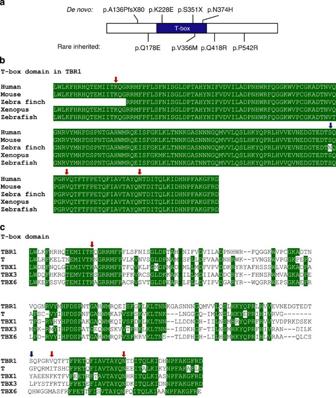Figure 1: TBR1 variants found in sporadic cases of ASD. (a) Schematic representation of TBR1 indicating changes found in sporadic ASD cases. (b) Sequence alignment of the T-box domains of TBR1 in human (UniProt accession Q16650), mouse (Q64336), zebra finch (deduced from genome sequence), xenopus (Q0IHV5) and zebrafish (B5DE34). (c) Sequence alignment of the T-box domains of human TBR1 (Q16650), T protein (O15178), TBX1 (O43435), TBX3 (O15119), TBX6 (O95947). Conserved residues are highlighted in green. Red arrows indicate residues mutated in sporadic ASD cases. The blue arrow indicates the first residue absent in the truncated S351X variant. 1a and Table 1 and Supplementary Table 1 ) [3] , [8] . No homozygous or compound heterozygous mutations in TBR1 were observed, consistent with murine knockout models, which show neonatal lethality [22] . However, there were several instances of heterozygous rare variants inherited from an unaffected parent. Such mutations could represent risk factors for ASD (for example, in combination with other mutations in the genomic background) [29] . Figure 1: TBR1 variants found in sporadic cases of ASD. ( a ) Schematic representation of TBR1 indicating changes found in sporadic ASD cases. ( b ) Sequence alignment of the T-box domains of TBR1 in human (UniProt accession Q16650), mouse (Q64336), zebra finch (deduced from genome sequence), xenopus (Q0IHV5) and zebrafish (B5DE34). ( c ) Sequence alignment of the T-box domains of human TBR1 (Q16650), T protein (O15178), TBX1 (O43435), TBX3 (O15119), TBX6 (O95947). Conserved residues are highlighted in green. Red arrows indicate residues mutated in sporadic ASD cases. The blue arrow indicates the first residue absent in the truncated S351X variant. Full size image Table 1 Description of TBR1 mutations found in ASD. Full size table Among the de novo mutations, the K228E and N374H mutations involve amino-acid substitutions at highly conserved positions within the T-box domain, which is involved in DNA-binding and protein–protein interactions ( Fig. 1b,c ). These mutations may therefore disturb these functions. The A136PfsX80 and S351X mutations are predicted to yield truncated proteins missing all or part of the T-box, which are unlikely to retain DNA-binding capacity. For the A136PfsX80 variant, the additional 80 amino acids following the frameshift do not show significant homology to known protein domains, but do alter the pI of TBR1 (pI of wild-type (WT) protein=6.9, pI of A136PfsX80=8.9). All four mutations are suspected to be causal due to their de novo occurrence coupled with in silico predictions of functional significance. In this study, we undertook empirical assessment of the impact of these mutations on protein function. Of the missense TBR1 mutations that were inherited from an unaffected parent, we selected three—Q178E, Q418R and P542R—for functional characterization based on the phenotype of affected probands and/or predicted deleterious effects on protein function ( Fig. 1a and Table 1 and Supplementary Table 1 ). A fourth mutation, V356M, was also chosen that was previously identified through a targeted TBR1 screen in a family with an ASD-affected sib-pair [30] and is found within the T-box ( Fig. 1b,c ). De novo TBR1 mutations disrupt protein cellular localization The expression levels of WT and mutant TBR1 proteins were assessed by western blotting of lysates from transfected cells ( Fig. 2a,b and Supplementary Fig. 1 ). WT TBR1 was detected at ~78 kDa. Protein variants arising from de novo and inherited missense mutations were of identical molecular weight and expressed in similar amounts to the WT protein, with the exception of K228E, which showed increased expression. The A136PfsX80 variant yielded a severely truncated product of only ~27 kDa and was expressed in higher levels compared with WT TBR1. In contrast, the S351X variant showed reduced expression and yielded a truncated protein of ~43 kDa. 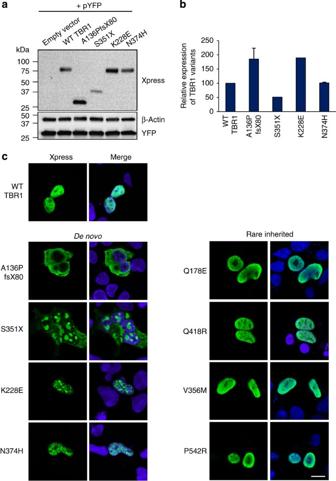Figure 2: Functional characterization of TBR1 protein variants identified in ASD. (a) Immunoblotting of whole-cell lysates from HEK293 cells co-transfected with TBR1 variants in pcDNA4.HisMax and an empty pYFP plasmid as a control for testing transfection efficiency. The expected molecular weights for the TBR1 proteins are: ~78 kDa=WT TBR1, K228E, N374H; ~27 kDa=A136PfsX80; ~43 kDa=S351X. (b) Relative expression of TBR1 variant proteins as determined by densitometric analysis of western blot data (average of two independent experiments±s.e.m.). (c) Immunofluorescence staining of HEK293 cells transfected with TBR1 variants. Xpress-tagged TBR1 proteins are shown in green. Nuclei were stained with Hoechst 33342 (blue). Scale bars=10 μm. Concordant results were seen in SHSY5Y cells, as shown inSupplementary Fig. 2. Figure 2: Functional characterization of TBR1 protein variants identified in ASD. ( a ) Immunoblotting of whole-cell lysates from HEK293 cells co-transfected with TBR1 variants in pcDNA4.HisMax and an empty pYFP plasmid as a control for testing transfection efficiency. The expected molecular weights for the TBR1 proteins are: ~78 kDa=WT TBR1, K228E, N374H; ~27 kDa=A136PfsX80; ~43 kDa=S351X. ( b ) Relative expression of TBR1 variant proteins as determined by densitometric analysis of western blot data (average of two independent experiments±s.e.m.). ( c ) Immunofluorescence staining of HEK293 cells transfected with TBR1 variants. Xpress-tagged TBR1 proteins are shown in green. Nuclei were stained with Hoechst 33342 (blue). Scale bars=10 μm. Concordant results were seen in SHSY5Y cells, as shown in Supplementary Fig. 2 . Full size image Subcellular localization of TBR1 protein variants was examined in transfected HEK293 cells by immunocytochemistry ( Fig. 2c ). Consistent with its role as a transcription factor, WT TBR1 localized to the nucleus and was excluded from nucleoli. Strikingly, all the de novo protein variants exhibited aberrant subcellular localization, consistent with loss-of-function. The A136PfsX80 variant exhibited a diffuse distribution in the cytoplasm and occasionally also in the nucleus. The S351X variant showed diffuse cytoplasmic distribution as well as large aggregates throughout the cell. The K228E and N374H variants retained import into the nucleus but a fraction formed abnormal aggregates. In contrast to the de novo mutants, all the variants arising from inherited mutations exhibited similar localization to the WT protein. Similar results were obtained when examining the subcellular localization of TBR1 variant proteins in transfected human neuroblastoma SHSY5Y cells ( Supplementary Fig. 2 ). Truncating TBR1 mutations abolish transcriptional repression TBR1 can function as both an activator and repressor of transcription [31] , [32] . TBR1-mediated repression of Fezf2 in layer 6 corticothalamic projection neurons restricts the origin of the corticospinal tract to layer 5, and murine Tbr1 is able to repress transcription in luciferase reporter assays through direct binding to a conserved consensus element found near Fezf2 (ref. 32 ). We demonstrated that human TBR1, which is 99.3% identical to the mouse protein and has an identical T-box ( Fig. 1b ), was also able to repress transcription from a luciferase reporter plasmid containing this element (a decrease of 56±2%; P< 0.001) ( Fig. 3 ). 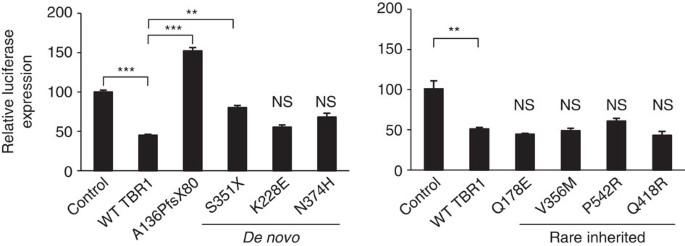Figure 3:De novo TBR1truncating mutations abolish transcriptional repression activity. Luciferase reporter assays for transcriptional regulatory activity of TBR1 variants in HEK293 cells. Values are expressed relative to the control. (***P<0.001, **P<0.01; NS, not significant when compared with WT TBR1). The mean±s.e.m. of three independent experiments performed in triplicate is shown. Figure 3: De novo TBR1 truncating mutations abolish transcriptional repression activity. Luciferase reporter assays for transcriptional regulatory activity of TBR1 variants in HEK293 cells. Values are expressed relative to the control. (*** P <0.001, ** P <0.01; NS, not significant when compared with WT TBR1). The mean±s.e.m. of three independent experiments performed in triplicate is shown. Full size image Both truncated TBR1 variants arising from de novo mutations demonstrated significant loss of repressive ability ( P< 0.001 and P< 0.01 respectively; Fig. 3 ), consistent with the total or partial loss of the T-box in these variants. Moreover, the A136PfsX80 variant resulted in increased reporter expression compared with cells transfected with an empty expression vector ( P< 0.001). This observation may be due to aberrant protein–protein interactions involving the new section of polypeptide resulting from the frameshift mutation, especially given the high expression level of the protein. In contrast to the truncated variants, the K228E and N374H variants did not differ significantly from WT TBR1 in their ability to repress transcription, suggesting that they at least partially retain DNA-binding capacity despite amino-acid changes within the T-box. In our functional analyses of the inherited missense mutations (of which only the V356M variant represents an amino-acid change within the T-box), no variant showed a significant difference in repressive ability compared with the WT protein ( Fig. 3 ). Thus, according to this assay, such mutations do not affect DNA-binding or transcriptional repression capabilities. Truncating mutations disrupt TBR1–CASK interaction Interaction partners of TBR1 remain largely unknown—the only protein reported to interact directly with TBR1 in the developing cerebral cortex is CASK, a membrane-associated guanylate kinase with roles in neural development and synaptic function [31] . Heterozygous mutations disrupting CASK have been reported in patients with severe intellectual disability (ID) and ASD [4] , [33] . Interaction between the T-box and carboxy terminal region of TBR1 and the guanylate kinase domain of CASK triggers redistribution of CASK from the plasma membrane to the nucleus, where it cooperates in the regulation of TBR1 target genes [31] , [34] . Accordingly, in our experiments, co-expression of CASK with WT TBR1 in HEK293 cells resulted in translocation of CASK to the nucleus and extensive co-localization of TBR1 with CASK ( Fig. 4a ). In contrast, co-expression of CASK with the truncated TBR1 variants resulting from de novo mutations revealed a lack of CASK redistribution and loss of TBR1/CASK co-localization ( Fig. 4b ). These findings are consistent with the mapping of the CASK-binding site within the C-terminal region of TBR1 (ref. 31 ). Intriguingly, CASK co-localizes in nuclear aggregates with the K228E and N374H TBR1 variants, suggesting that these mutants continue to interact with CASK and could thereby trigger aberrant localization of CASK within neurons ( Fig. 4c ). The amino-acid changes in TBR1 resulting from inherited missense mutations do not disrupt recruitment of CASK into the nucleus ( Supplementary Fig. 3 ). The effects of the TBR1 variant proteins on CASK localization were validated in transfected SHSY5Y cells ( Supplementary Fig. 4 ). Although three of the mutations (V356M, Q418R, P542R) lie within the known CASK-binding region, our findings suggest that these amino acids are not crucial for CASK–TBR1 interaction. 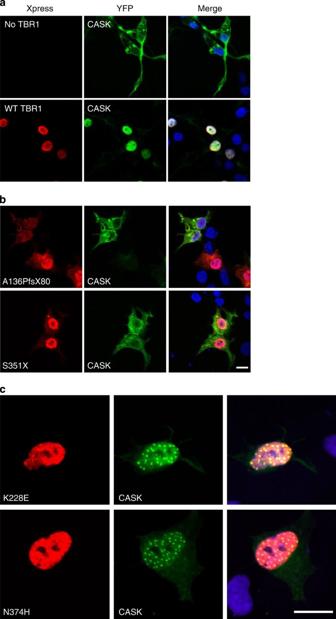Figure 4:De novotruncating TBR1 mutations disrupt interactions with CASK. Fluorescence micrographs of HEK293 cells co-transfected with CASK and (a) WT TBR1, (b)de novotruncating variants and (c)de novomissense variants. Xpress-tagged TBR1 proteins are shown in red (left-hand side), whereas CASK fused to YFP is shown in green (middle). Nuclei were stained with Hoechst 33342 (blue). Scale bars fora–c=10 μm. Concordant results were seen in SHSY5Y cells, as shown inSupplementary Fig. 4. Figure 4: De novo truncating TBR1 mutations disrupt interactions with CASK. Fluorescence micrographs of HEK293 cells co-transfected with CASK and ( a ) WT TBR1, ( b ) de novo truncating variants and ( c ) de novo missense variants. Xpress-tagged TBR1 proteins are shown in red (left-hand side), whereas CASK fused to YFP is shown in green (middle). Nuclei were stained with Hoechst 33342 (blue). Scale bars for a – c =10 μm. Concordant results were seen in SHSY5Y cells, as shown in Supplementary Fig. 4 . Full size image TBR1 forms homodimers Homodimerization has been observed in a subset of T-box transcription factors, and in some cases is required for binding to palindromic DNA sites [35] . To determine whether TBR1 can form homodimers, we used the bioluminescence resonance energy transfer (BRET) assay, a method for monitoring protein–protein interactions in live cells [36] . In this assay, a protein of interest is expressed as a fusion protein with Renilla luciferase (donor), and its putative interaction partner as a fusion protein with YFP (acceptor). An interaction between the two proteins may bring the luciferase and YFP moieties sufficiently close for non-radiative energy transfer to occur, causing a measurable shift in the wavelength of the emitted light (the BRET signal). When YFP–TBR1 and luciferase–TBR1 fusion proteins were co-expressed in cells, a significant increase in BRET signal was observed compared with when YFP–TBR1 was expressed with a control (nuclear-targeted) luciferase, suggesting that TBR1 is able to homodimerize ( Fig. 5a ). We confirmed that the fusion proteins were correctly localized in the cell ( Supplementary Fig. 5 ). 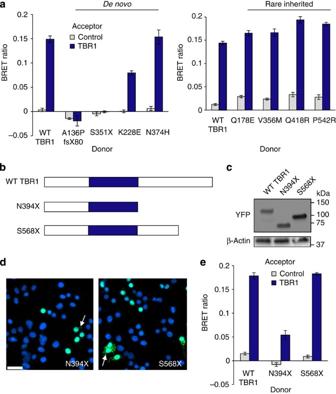Figure 5: TBR1 homodimerizes. (a) BRET assays for interaction between WT and mutant TBR1 proteins. (b) Schematic representation of synthetic TBR1 variants. (c) Immunoblot of YFP–TBR1 fusion proteins in transfected HEK293 cells. (d) Fluorescence microscopy images of HEK293 cells transfected with synthetic TBR1 variants fused to YFP (shown in green). Nuclei were stained with Hoechst 33342 (blue). Arrows indicate protein in the cytoplasm. Scale bar, 20 μm. Concordant results were seen in SHSY5Y cells, as shown inSupplementary Fig. 2. (e) BRET assays for interaction between WT TBR1 and synthetic truncations. Foraandebars represent the mean corrected BRET ratios±s.e.m. of one experiment performed in triplicate. BRET assays were performed in HEK293 cells. Figure 5: TBR1 homodimerizes. ( a ) BRET assays for interaction between WT and mutant TBR1 proteins. ( b ) Schematic representation of synthetic TBR1 variants. ( c ) Immunoblot of YFP–TBR1 fusion proteins in transfected HEK293 cells. ( d ) Fluorescence microscopy images of HEK293 cells transfected with synthetic TBR1 variants fused to YFP (shown in green). Nuclei were stained with Hoechst 33342 (blue). Arrows indicate protein in the cytoplasm. Scale bar, 20 μm. Concordant results were seen in SHSY5Y cells, as shown in Supplementary Fig. 2 . ( e ) BRET assays for interaction between WT TBR1 and synthetic truncations. For a and e bars represent the mean corrected BRET ratios±s.e.m. of one experiment performed in triplicate. BRET assays were performed in HEK293 cells. Full size image All de novo and inherited variants carrying single amino-acid changes retained the ability to dimerize with themselves and with WT TBR1 in the BRET assay ( Fig. 5a and Supplementary Fig. 6a ). Strikingly, co-expression of WT TBR1 and variants resulting from de novo missense mutations (K228E, N374H) resulted in extensive co-localization of WT and mutant proteins in nuclear aggregates (see Supplementary Fig. 6b ). Given that the mutations occur in the heterozygous state in ASD cases, it is possible that these TBR1 variants exert a dominant-negative effect by interfering with functions of WT TBR1. In contrast, the truncated proteins resulting from de novo mutations showed a complete loss of interaction with WT TBR1 and a lack of self-association ( Fig. 5a and Supplementary Fig. 6a ). Loss of interaction with WT protein may be due to the aberrant subcellular localization of the truncated proteins; however, the absence of self-association suggests that the T-box and/or C-terminal region of TBR1 may be important for homodimerization. To test this hypothesis, we created two truncated TBR1 proteins, N394X and S568X, which lack portions of the C-terminal region but retain the complete T-box ( Fig. 5b ). Expression of YFP-fusion proteins containing these two variants was examined by western blotting and fluorescence microscopy ( Fig. 5c,d and Supplementary Fig. 2b ), which revealed that both variants are predominantly nuclear but are also occasionally found in cytoplasmic aggregates. The BRET assay showed that the S568X variant, which lacks the final 114 residues, can interact with itself and with full-length TBR1 to a similar degree as the WT protein, whereas the N394X variant, which lacks the final 288 residues following the T-box, shows a reduced ability to associate with itself and with full-length TBR1 ( Fig. 5e and Supplementary Fig. 6c ), indicating that the 394–568 region is important for homodimerization. Homodimerization of the N394X synthetic variant was still greater than the S351X variant found in ASD, suggesting that the T-box is sufficient for some homodimerization to occur, consistent with previous studies [37] . Further experiments will be required to pinpoint the region(s) within the C terminus of TBR1 that are involved in dimerization, and to determine if the C-terminal region is capable of self-association in absence of the T-box. TBR1 interacts with the FOXP2 transcription factor A prior yeast two-hybrid screen suggested TBR1 as a putative interactor of the FOXP2 transcription factor [19] . Rare disruptions of FOXP2 are implicated in a speech/language disorder, involving developmental verbal dyspraxia accompanied by impairments in expressive and receptive language [20] , [38] , [39] . Thus, an interaction between TBR1 and FOXP2 could represent a molecular link between distinct neurodevelopmental disorders involving language deficits. We used the BRET assay to analyse the interaction of TBR1 with three naturally occurring FOXP2 isoforms found in the brain [38] , [40] ( Fig. 6a ). The canonical FOXP2 isoform (isoform I) was able to interact with TBR1, as was isoform III, which lacks the first 92 amino acids ( Fig. 6b ). Isoform 10+, which lacks the C-terminal region of FOXP2 spanning the DNA-binding domain, showed a complete loss of interaction with TBR1 ( Fig. 6b ). While FOXP2 isoforms I and III are nuclear, isoform 10+ is localized to the cytoplasm, which may account for its lack of interaction with WT TBR1 ( Fig. 6c and Supplementary Fig. 7 ). Alternatively, the C-terminal region of FOXP2 may be involved in the interaction. 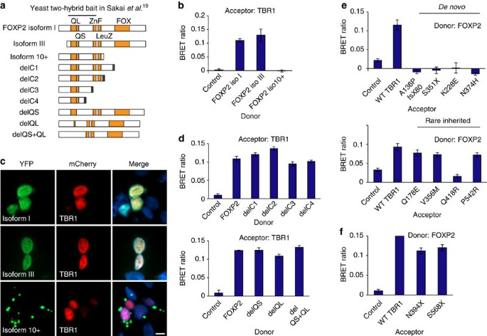Figure 6: TBR1 interacts with FOXP2 through the T-box domain. (a) Schematic representation of recombinant FOXP2 proteins used in BRET assays. FOXP2 contains long (QL) and short (QS) polyglutamine tracts, and zinc finger (ZnF), leucine zipper (LeuZ) and FOX DNA-binding domains. Isoforms I, III and 10+ represent natural isoforms, other constructs are synthetic. A nuclear-targeting signal appended to the C terminus in variants delC1-delC4 is indicated in black. The putative TBR1-binding region based on yeast two-hybrid data19is also shown. (b) BRET assays for interaction between WT TBR1 and naturally occurring FOXP2 isoforms. (c) Fluorescence images of HEK293 cells co-transfected with TBR1 and FOXP2 variants. FOXP2 variants fused to YFP are shown in green (left-hand side), whereas TBR1 fused to mCherry is shown in red (middle). Nuclei were stained with Hoechst 33342 (blue). Scale bar, 5 μm. Concordant results were seen in SHSY5Y cells, as shown inSupplementary Fig. 7. (d) BRET assays for interaction between WT TBR1 and synthetic FOXP2 variants. (e) BRET assays for interaction between WT FOXP2 and TBR1 variants found in ASD. (f) BRET assays for interaction between WT FOXP2 and synthetic TBR1 truncations. Inb,d–f, bars represent the corrected mean BRET ratios±s.e.m. of one experiment performed in triplicate. BRET assays were performed in HEK293 cells. Figure 6: TBR1 interacts with FOXP2 through the T-box domain. ( a ) Schematic representation of recombinant FOXP2 proteins used in BRET assays. FOXP2 contains long (QL) and short (QS) polyglutamine tracts, and zinc finger (ZnF), leucine zipper (LeuZ) and FOX DNA-binding domains. Isoforms I, III and 10+ represent natural isoforms, other constructs are synthetic. A nuclear-targeting signal appended to the C terminus in variants delC1-delC4 is indicated in black. The putative TBR1-binding region based on yeast two-hybrid data [19] is also shown. ( b ) BRET assays for interaction between WT TBR1 and naturally occurring FOXP2 isoforms. ( c ) Fluorescence images of HEK293 cells co-transfected with TBR1 and FOXP2 variants. FOXP2 variants fused to YFP are shown in green (left-hand side), whereas TBR1 fused to mCherry is shown in red (middle). Nuclei were stained with Hoechst 33342 (blue). Scale bar, 5 μm. Concordant results were seen in SHSY5Y cells, as shown in Supplementary Fig. 7 . ( d ) BRET assays for interaction between WT TBR1 and synthetic FOXP2 variants. ( e ) BRET assays for interaction between WT FOXP2 and TBR1 variants found in ASD. ( f ) BRET assays for interaction between WT FOXP2 and synthetic TBR1 truncations. In b , d – f , bars represent the corrected mean BRET ratios±s.e.m. of one experiment performed in triplicate. BRET assays were performed in HEK293 cells. Full size image To locate the TBR1-binding site within FOXP2, we created a series of four C-terminal deletions in FOXP2 ( Fig. 6a ). A nuclear-targeting signal was appended to the C terminus of these truncated proteins, which lack endogenous nuclear-targeting signals. All these truncated proteins retained the ability to interact with TBR1 in the BRET assay ( Fig. 6d ), indicating that the TBR1-binding site lies within the N-terminal 258 residues of FOXP2. In the yeast two-hybrid screen which suggested TBR1 interaction, a region of FOXP2 encompassing residues 122–382 was used as the bait protein [19] . Together, these findings suggest that the TBR1-binding site lies within region 122–258 of the canonical FOXP2 isoform. This region includes two polyglutamine (polyQ) tracts that are not present in other FOXP family members. We generated FOXP2 variants that lacked one or both polyQ tracts ( Fig. 6a ). All three variants retained the ability to interact with TBR1 ( Fig. 6d ), indicating that the polyQ tracts are not required for this interaction. We also tested the interaction between TBR1 and two neurally expressed FOXP2 paralogs, FOXP1 and FOXP4, which have Q-rich domains but lack polyQ tracts ( Supplementary Fig. 8 ). In the BRET assay, both FOXP1 and FOXP4 were able to interact with TBR1, confirming our observations with the synthetic FOXP2 polyQ-deletion constructs. We conclude that TBR1 binding is likely to involve the regions flanking or between the two polyglutamine tracts that are conserved in FOXP1 and FOXP4. In agreement with these results, TBR1–FOXP2 interaction was not disrupted by an in-frame deletion of E400 in FOXP2 ( Supplementary Fig. 8 ), a residue which is known to be important for FOXP2 homodimerization [41] . An intact T-box is required for TBR1–FOXP2 interaction Next, we investigated the effects of de novo and inherited TBR1 mutations on interaction with FOXP2 ( Fig. 6e ). All four de novo mutations abolished interactions with FOXP2. In contrast, three TBR1 variants arising from inherited missense mutations (Q178E, V356M and P542R) showed BRET signals comparable with those seen with WT TBR1. Interestingly, the inherited Q418R variant demonstrated reduced interaction with FOXP2. This observation cannot be attributed to differential expression or aberrant subcellular localization of the mutant protein. The synthetic truncated TBR1 variants, both of which retain an intact T-box, were still able to interact with FOXP2 ( Fig. 6f ). Together, these data suggest that the T-box domain is mediating the TBR1–FOXP2 interaction. Aetiological FOXP2 mutations disrupt interaction with TBR1 Finally, we investigated if the TBR1–FOXP2 interaction was affected by two different pathogenic FOXP2 point mutations, each known to cause a rare monogenic speech and language disorder ( Fig. 7a ). The R553H mutation yields a substitution at a key residue in the DNA-binding domain of FOXP2, and was identified as the result of linkage mapping in a large multigenerational pedigree, the KE family [38] , [42] . The R328X mutation introduces a premature stop codon to yield a protein product lacking the leucine zipper dimerization domain and the DNA-binding domain, and was discovered through targeted FOXP2 screening [43] . Both mutations severely disrupt protein function [44] . Strikingly, both R553H and R328X mutations interfere with the ability of FOXP2 to interact with TBR1 ( Fig. 7b ). For the R328X variant, this loss of interaction with TBR1 may be largely due to cytoplasmic mislocalization of FOXP2 ref. 44 ( Fig. 7c and Supplementary Fig. 7 ), since a comparable fragment of the protein did interact with TBR1 when artificially directed to the nucleus ( Fig. 6d ). The reduced interaction observed with the R553H variant may also relate to its partial mislocalization to the cytoplasm or protein aggregation [44] ( Fig. 7c and Supplementary Fig. 7 ). 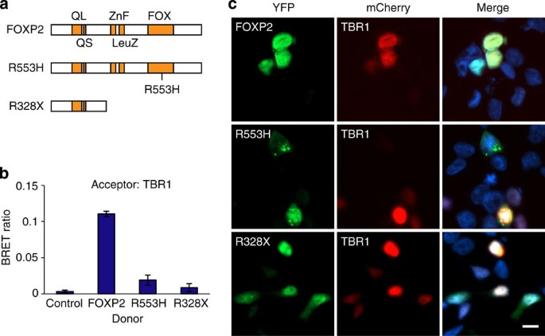Figure 7: FOXP2 variants found in speech/language disorders do not interact with TBR1. (a) Schematic representation of FOXP2 variants found in speech/language disorders. (b) BRET assays for interaction of WT TBR1 with FOXP2 variants. (c) Fluorescence images of HEK293 cells co-transfected with TBR1 and FOXP2 variants. FOXP2 variants fused to YFP are shown in green (left-hand side), whereas TBR1 fused to mCherry is shown in red (middle). Nuclei were stained with Hoechst 33342 (blue). Scale bar, 10 μm. Concordant results were seen in SHSY5Y cells, as shown inSupplementary Fig. 7. Inb, bars represent the corrected mean BRET ratios±s.e.m. of one experiment performed in triplicate. BRET assays were performed in HEK293 cells. Figure 7: FOXP2 variants found in speech/language disorders do not interact with TBR1. ( a ) Schematic representation of FOXP2 variants found in speech/language disorders. ( b ) BRET assays for interaction of WT TBR1 with FOXP2 variants. ( c ) Fluorescence images of HEK293 cells co-transfected with TBR1 and FOXP2 variants. FOXP2 variants fused to YFP are shown in green (left-hand side), whereas TBR1 fused to mCherry is shown in red (middle). Nuclei were stained with Hoechst 33342 (blue). Scale bar, 10 μm. Concordant results were seen in SHSY5Y cells, as shown in Supplementary Fig. 7 . In b , bars represent the corrected mean BRET ratios±s.e.m. of one experiment performed in triplicate. BRET assays were performed in HEK293 cells. Full size image We report the first functional characterization of TBR1 mutations identified in individuals with sporadic ASD ( Table 2 ). We found that the de novo mutations studied here disrupted one or more of the aspects of protein function tested, whereas TBR1 mutations inherited from unaffected parents had little or no impact on protein function. These findings provide empirical support for the effectiveness of focusing on de novo mutation events for understanding the biology underlying sporadic cases of severe neurodevelopmental disorders. Moreover, we showed that TBR1 interacts with FOXP2, a regulatory factor implicated in speech/language disorder, demonstrating that this interaction is disrupted by pathogenic mutations in either protein, suggesting a molecular link between distinct neurodevelopmental disorders. Table 2 Summary of functional investigations of TBR1 variants found in ASD. Full size table Two of the de novo mutations studied here are single-nucleotide indels that introduce premature termination codons into the coding sequence. These mutations occur before the final exon boundary and may trigger nonsense-mediated decay. However, the degradation of mutated TBR1 transcripts in patient cells cannot be assessed due to the absence of TBR1 expression in peripheral tissues. The analyses of protein function described here indicate that any truncated protein that is produced is non-functional, since the protein exhibits loss of nuclear localization, loss of interaction with the co-activator CASK and deficiency in transcriptional repression activity. Coupled with the observation that the truncated proteins cannot dimerize with WT TBR1, it seems likely that the pathogenic mechanism of these mutations is haploinsufficiency. This hypothesis is supported by the discovery of heterozygous de novo microdeletions encompassing TBR1 in probands with developmental delay, ASD and ID [45] , [46] , [47] . Furthermore, anatomical and behavioural characterization of heterozygous Tbr1 mice revealed that loss of one Tbr1 allele impairs amygdalar axonal projections and results in cognitive abnormalities [48] . Two of the four de novo TBR1 mutations are missense mutations within the T-box. The amino-acid residues affected by the K228E and N374H mutations are conserved in T-box sequences from divergent proteins ( Fig. 1b,c ), indicating that they are likely to be important for the functioning of this domain. These mutations showed more moderate effects on protein function than those resulting in truncated TBR1 protein. They did not abolish nuclear import or transcriptional repression activity in our assays, but were found to aggregate in the nucleus. It is possible that subtle effects conferred by these variants, not evident from in vitro experiments, may be important in vivo . Interestingly, it was recently shown that the overexpression of N374H in cultured amygdalar neurons from heterozygous Tbr1 mice fails to rescue the axon outgrowth defect observed in these neurons, whereas overexpression of WT TBR1 restored normal axonogenesis [48] . In our experiments, K228E and N374H were no longer able to interact with either the co-activator CASK or transcription factor FOXP2 (see below) suggesting that regulation of different TBR1 target genes may be selectively affected by these mutations, with particular dysregulation of genes that are regulated by the TBR1–CASK complex, and/or co-regulated by FOXP2. It is tempting to speculate that CASK and/or FOXP2 might be involved in TBR1-mediated axonogenesis. Crystal structures of the T-box domains from human TBX3 and Xenopus laevis Xbra show that the residue equivalent to K228 makes direct contact with the DNA backbone in Xbra, but not in TBX3, while the residues equivalent to N374 do not make direct contact with DNA in either structure [35] , [49] . Thus, the missense mutations observed in ASD probands may not completely abolish DNA-binding activity, consistent with the retention of transcriptional repression activity presented here, but could have milder effects on the affinity or specificity of DNA recognition, or on protein stability. A crystal structure of TBR1 bound to DNA would help clarify the role of these residues in DNA recognition. The K228E and N374H variants retained the ability to dimerize with WT TBR1, causing the WT protein to become localized to nuclear aggregates. Thus, the pathogenic mechanism of these mutations may include a dominant-negative effect that reduces the effective dosage of WT protein. Overall, our data suggest that mutations that lead to a reduction in the amount of functional TBR1 protein are causative in sporadic cases of ASD. It is intriguing that there were variable effects among these different causative mutations—aetiological missense mutations within the DNA-binding domain did not have as dramatic an effect on TBR1 protein function as the truncating mutations in our assays. These findings are in line with the expected odds ratio for these particular classes of mutation. Interestingly, the severity of cognitive deficits in individuals carrying TBR1 mutations may reflect the severity of the disruption to protein function. The ASD cases carrying truncating mutations have mild-to-moderate ID, whereas those with missense mutations have milder cognitive impairments ( Supplementary Table 1 : non-verbal IQ scores: 41=A136PfsX80; 63=S351X; 78=K228E; 74=N374H). Our functional characterization of TBR1 mutations supports the hypothesis that de novo mutations with highly deleterious effects on protein function are an important cause of severe sporadic ASD. With the exception of Q418R (see below), none of the inherited variants displayed significant effects on protein function in our assays. While it remains possible that subtle effects on protein function went undetected in these analyses, overall our data do not support a contributory role for inherited TBR1 mutations in sporadic ASD. In addition to characterizing TBR1 mutants found in ASD, we also investigated the interaction of TBR1 with the language-related transcription factor FOXP2. We confirmed an interaction between these proteins and demonstrated that this interaction involves the T-box of TBR1. Previous studies also highlighted the role of the T-box in protein–protein interactions, such as between TBR1 and CASK [31] and between TBX5 and NKX2.5 (ref. 50 ). The TBR1-binding site within FOXP2 was mapped to the regions flanking the two polyQ tracts, a part of the protein with no established function. The interaction between TBR1 and FOXP2 is likely to be physiologically relevant due to temporal and spatial overlap in expression of the two genes in several brain areas, including layer 6 glutamatergic corticothalamic projection neurons [21] , [22] , [23] , [51] , [52] . It will be interesting in future to identify the specific developmental stages and neuronal subtypes in which TBR1–FOXP2 interactions occur. Individuals with mutations in either TBR1 or FOXP2 exhibit speech and language deficits, with the ASD probands showing language delay and regression. Therefore, it is interesting that the TBR1–FOXP2 interaction is disrupted both by de novo TBR1 mutations in ASD probands and by FOXP2 mutations found in patients with a primary speech and language disorder (in the absence of autism). Loss of TBR1–FOXP2 interaction may therefore contribute to speech and language deficits in the context of two distinct neurodevelopmental disorders. Intriguingly, the interaction was also disrupted by the Q418R inherited mutation, which is predicted to be benign ( Table 1 ). The lack of interaction between this mutant and FOXP2 may contribute to the discrepancy between non-verbal IQ (86) and verbal IQ (58) scores in this proband ( Supplementary Table 1 ). The importance of the TBR1–FOXP2 interaction to normal speech and language development may lie in the co-regulation of gene expression by these two transcription factors. The ASD-susceptibility gene AUTS2 is a good candidate for co-regulation by TBR1 and FOXP2. AUTS2 is a known TBR1 target [53] and in expression profiling of human cells with inducible FOXP2 expression, upregulation of AUTS2 was one of the most significant changes associated with induction of FOXP2 expression (P.D. and S.E.F., unpublished data). In summary, our findings highlight the power of coupling novel genetic findings with empirical data to flesh out more comprehensive molecular networks. By performing functional characterization of de novo and rare inherited TBR1 mutations found in sporadic ASD, we identified novel protein characteristics, such as TBR1 homodimerization, and built on existing protein–protein networks with new interactions, at the same time providing mechanistic bridges between neurodevelopmental disorders ( Fig. 8 ). Next-generation screens of larger ASD cohorts are set to reveal additional de novo mutations in candidates including TBR1 , GRIN2B , RELN and AUTS2 —genes that are recurrently mutated and belong to shared molecular networks. Without experimental validation, such data sets will most likely remain biologically uninformative. The functional assays established here can be used to systematically investigate effects of novel mutations disrupting members of this pathway. At present, the lack of high-throughput testing of multiple genetic variants hinders the extrapolation of such assays to the clinic for diagnostic purposes. Development of such multiplex methods is underway [25] . Coupled with strong genetic predictors, such as de novo variants, this will undoubtedly aid in robustly defining the molecular networks that go awry in ASD. 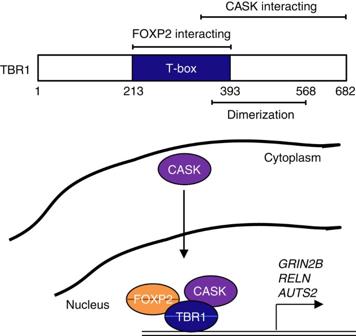Figure 8: Novel insights into TBR1-related molecular networks underlying sporadic ASD. By interacting with CASK, TBR1 regulates several ASD candidate genes, such asGRIN2B,AUTS2andRELN—all of which are recurrently mutated in ASD. In areas of the brain with overlapping expression patterns, such as in glutamatergic layer 6 neurons, the TBR1–FOXP2 interaction may result in co-ordinated regulation of common downstream targets. Figure 8: Novel insights into TBR1-related molecular networks underlying sporadic ASD. By interacting with CASK, TBR1 regulates several ASD candidate genes, such as GRIN2B , AUTS2 and RELN— all of which are recurrently mutated in ASD. In areas of the brain with overlapping expression patterns, such as in glutamatergic layer 6 neurons, the TBR1–FOXP2 interaction may result in co-ordinated regulation of common downstream targets. Full size image Identification of TBR1 variants De novo and rare inherited mutations were previously identified through whole exome or targeted resequencing [3] , [6] , [8] . Cell culture and transfection HEK293 and SHSY5Y cell lines were obtained from ECACC (catalogue numbers: 85120602 for HEK293 and 94030304 for SHSY5Y). HEK293 cells were grown in Dulbecco’s modified Eagle’s medium and SHSY5Y cells in DMEM-F12 (Invitrogen). Media were supplemented with 10% fetal bovine serum (Invitrogen). Transfections were performed using GeneJuice (Merck-Millipore). DNA expression constructs and site-directed mutagenesis pcDNA4.HisMax.TBR1, pcDNA4.HisMax.A136PfsX80 and pJET1.2.CASK were synthesized by GenScript USA. S351X, K228E, N374H, Q178E, V356M, Q418R and P542R TBR1 variants were generated using the pcDNA4.HisMax.TBR1 as template with the QuikChange II Site-Directed Mutagenesis Kit (Agilent) (primer sequences are listed in Supplementary Table 2 ). Synthetic TBR1 truncation variants were PCR amplified (N394X: Fwd 5′-GAATTCATGCAGCTGGAGCACTGCCTT-3′, Rev 5′-TCTAGATTAATCCCGAAATCCTTTTGC-3′; S568X: Fwd 5′-GAATTCATGCAGCTGGAGCACTGCCTT-3′, Rev 5′- TCTAGATTAGTTGGGCCAGCAGGGCAG-3′) and cloned into pCR2.1-TOPO (Invitrogen). TBR1 cDNAs were subcloned using Eco RI/ Xba I restriction sites into a modified pmCherry-C1 vector (Clontech), as well as pLuc and pYFP expression vectors [36] . CASK cDNA was subcloned using Eco RI/ Kpn I restriction sites into the pYFP expression vector. FOXP variants were PCR amplified, cloned into pCR2.1-TOPO and subcloned using Bam HI/ Xba I restriction sites into pLuc and pYFP expression vectors (primer sequences are listed in Supplementary Table 3 ). The FOXP2.delQ variants were generated using a PCR-based strategy. The control plasmids pLuc-control and pYFP-control express the Renilla luciferase and YFP proteins with a C-terminal nuclear localization signal [36] . All constructs were verified by Sanger sequencing. SDS–PAGE and western blotting Cells were transfected with equimolar concentrations of TBR1 expression plasmids. Whole-cell lysates were extracted by treatment with lysis buffer (100 mM Tris pH 7.5, 150 mM NaCl, 10 mM EDTA, 0.2% Triton X-100, 1% PMSF, 1 × protease inhibitor cocktail; all from Sigma) for 10 min at 4 °C, before centrifuging at 10,000 g for 30 min at 4 °C to remove cell debris. Proteins were resolved on 4–15% Tris–Glycine gels and transferred onto polyvinylidene fluoride membranes. Membranes were probed with Invitrogen mouse anti-Xpress (for pcDNA4.HisMax constructs; 1:1,000) or Clontech mouse anti-EGFP (for pYFP constructs; 1:8,000) overnight at 4 °C, followed by incubation with HRP-conjugated goat anti-mouse IgG for 45 min at room temperature (Bio-Rad; 1:2,000). Proteins were visualized using Novex ECL Chemiluminescent Substrate Reagent Kit (Invitrogen) and the ChemiDoc XRS+ System (Bio-Rad). Equal protein loading was confirmed by stripping blots and reprobing using Sigma anti-β-actin antibody (1:10,000). Bands were quantified by densitometry using the Chemidoc XRS+ System image analysis software (Bio-Rad). A value for the transfection efficiency of TBR1 constructs was obtained by dividing the YFP signal by the β-actin signal. The relative expression of TBR1 variants was then derived by dividing the Xpress signal by the transfection efficiency. Immunofluorescence Cells were seeded onto coverslips coated with poly- L -lysine (Sigma) and 36 h post transfection, cells were fixed using 4% paraformaldehyde solution (Electron Microscopy Sciences) for 10 min at room temperature. Cells were stained with mouse anti-Xpress (1:500) followed by Alexa Fluor 488-conjugated goat anti-mouse IgG (H+L; 1:1,000) (both Invitrogen) to visualize proteins expressed from pcDNA4.HisMax. YFP and mCherry fusion proteins were visualized by direct fluorescence. Nuclei were visualized with Hoechst 33342 (Invitrogen). Fluorescence images were obtained using a LSM510 confocal microscope with LSM Image Software or an Axiovert A-1 fluorescent microscope with ZEN Image Software (Zeiss). Luciferase assays The pGL3-CMV firefly luciferase reporter plasmid including the Tbr1-binding site near Fezf2 was a kind gift of Prof. Sestan, Yale University [32] . Cells were transfected with 45 ng of firefly luciferase reporter construct, 5 ng of Renilla luciferase normalization control (pRL-TK; Promega) and 200 ng TBR1 expression construct (WT or mutant in pcDNA4.HisMax) or empty vector (pcDNA4.HisMax). Forty-eight hours post transfection, firefly luciferase and Renilla luciferase activities were measured in a TECAN F200PRO microplate reader using the Dual-Luciferase Reporter Assay system (Promega). BRET assay BRET assays were performed as described [36] . Briefly, cells were transfected with pairs of YFP and luciferase fusion proteins in 96-well plates. EnduRen (60 μM; Promega) was added to cells 36–48 h after transfection. Four hours later, emission readings (integrated over 10 s) were taken using a TECAN F200PRO microplate reader using the Blue1 and Green1 filter sets. Expression levels of the YFP-fusion proteins were monitored by taking fluorescence readings using the filter set and dichroic mirror suitable for green fluorescent protein (excitation 480 nm, emission 535 nm). The corrected BRET ratio was obtained as follows: [Green1 (experimental condition) /Blue1 (experimental condition) ]−[Green1 (control condition) /Blue1 (control condition) ]. The control proteins were Renilla luciferase and YFP fused to a C-terminal nuclear localization signal. The BRET assay setup, including the design of appropriate controls and data interpretation, is extensively discussed in Deriziotis et al. [36] Statistical significance The statistical significance of the luciferase reporter assays was analysed using a one-way analysis of variance and a Tukey’s post hoc test. How to cite this article : Deriziotis, P. et al. De novo TBR1 mutations in sporadic autism disrupt protein functions. Nat. Commun. 5:4954 doi: 10.1038/ncomms5954 (2014).